Roles of lymphatic endothelial cells expressing peripheral tissue antigens in CD4 T-cell tolerance induction Lymphatic endothelial cells (LECs) directly express peripheral tissue antigens and induce CD8 T-cell deletional tolerance. LECs express MHC-II molecules, suggesting they might also tolerize CD4 T cells. We demonstrate that when β-galactosidase (β-gal) is expressed in LECs, β-gal-specific CD8 T cells undergo deletion via the PD-1/PD-L1 and LAG-3/MHC-II pathways. In contrast, LECs do not present endogenous β-gal in the context of MHC-II molecules to β-gal-specific CD4 T cells. Lack of presentation is independent of antigen localization, as membrane-bound haemagglutinin and I-Eα are also not presented by MHC-II molecules. LECs express invariant chain and cathepsin L, but not H2-M, suggesting that they cannot load endogenous antigenic peptides onto MHC-II molecules. Importantly, LECs transfer β-gal to dendritic cells, which subsequently present it to induce CD4 T-cell anergy. Therefore, LECs serve as an antigen reservoir for CD4 T-cell tolerance, and MHC-II molecules on LECs are used to induce CD8 T-cell tolerance via LAG-3. Immune tolerance is imposed through multiple processes that begin during thymic T-cell development and continue in the periphery. During negative selection in the thymus, medullary thymic epithelial cells (mTECs) and dendritic cells (DCs) present self-antigens to tolerize auto-reactive T cells. Intrinsic tolerance mechanisms induce deletion or anergy of high-affinity self-reactive T cells, whereas lower affinity CD4 cells are converted into regulatory T cells (T reg ) that mediate extrinsic tolerance [1] , [2] . DCs can acquire antigen in the periphery and migrate into the thymus [3] , or thymic resident DCs can capture circulating antigen [4] . In addition to presenting ubiquitous antigens, mTECs also transcribe and present a variety of peripheral tissue antigens (PTAs) under the control of the autoimmune regulatory element (Aire) [5] , [6] , increasing the diversity of self-antigens presented in the thymus. Thymic tolerance does not eliminate all self-reactive T cells, necessitating mechanisms of peripheral tolerance. Immature DCs continually survey peripheral tissues to acquire self-antigens, which are presented in the draining lymph nodes (LNs) to induce T-cell deletion, anergy or T reg formation [7] . In contrast to DCs, which are specialized for acquiring antigens from other tissues, several subsets of LN cells transcribe PTAs, analogous to mTECs. Extrathymic Aire-expressing cells transcribe and present PTAs in an Aire-dependent manner, leading to CD8 T-cell deletional tolerance and CD4 T-cell anergy [8] , [9] . Extrathymic Aire-expressing cells are developmentally related to DCs [9] . PTAs are transcriptionally expressed independently of Aire by several subsets of radioresistant LN stromal cells (LNSCs), including lymphatic endothelial cells (LECs), fibroblastic reticular cells (FRCs) and blood endothelial cells (BECs) [10] , [11] . Although the effects of PTAs expressed in BECs have not been tested, LECs and FRCs both induce deletional tolerance of CD8 T cells [10] , [11] , [12] , [13] . We previously showed that LECs transcribe and present an epitope from the melanocyte differentiation protein tyrosinase, leading to proliferation and deletion of tyrosinase-specific CD8 T cells [10] , [14] . Proliferating tyrosinase-specific CD8 T cells activated by LECs in the absence of 4-1BB co-stimulation upregulate PD-1, which binds to PD-L1 on a radioresistant stromal cell, inhibits the upregulation of the IL-2 receptor and leads to death [12] . LECs express the highest level of PD-L1 among the LNSC. LECs also express herpesvirus entry mediator (HVEM) and major histocompatibility complex (MHC)-II [12] , which are ligands for the BTLA/CD160 and LAG-3 inhibitory pathways, respectively [15] . Tyrosinase and PD-L1 are more highly expressed by LECs in the LN (LN-LECs) compared with LECs from tissue lymphatics in the diaphragm or colon [16] , suggesting the LN microenvironment endows LN-LECs with tolerogenic properties not found in tissue LECs. In this study, we investigated whether MHC-II expression on LN-LECs is related to their tolerogenic role, and whether MHC-II is used to induce CD4 T-cell tolerance. The MHC-II antigen presentation pathway has been extensively studied in professional antigen-presenting cells (APC) and in cell lines. MHC-II molecules are synthesized in the ER and associated with invariant chain (Ii), which targets the complex into late endosomal MHC-II-loading compartments (MIICs). Next, Ii is cleaved by cathepsins, leaving the class II Ii-associated peptide (CLIP) in the peptide-binding groove. CLIP is exchanged for antigenic peptides by the non-classical MHC-II molecule H2-M. H2-M can be inhibited by H2-O, altering the representation of peptides presented [17] . LECs express MHC-II [12] , but the ability of LECs to load and present self-peptides on MHC-II molecules has not been investigated. In addition, it is unknown whether PTA expression in LECs leads to CD4 T-cell tolerance. To investigate whether LECs present PTAs on MHC-II molecules and induce CD4 T-cell tolerance, we created transgenic systems where the model antigens β-galactosidase (β-gal) or haemagglutinin (HA) are expressed in LECs under the control of LEC-specific Lyve-1 or Prox1 promoters. Using these complementary models, we demonstrate that LECs do not directly present these PTAs on MHC-II molecules, but instead provide antigen to DCs to induce CD4 T-cell anergy. LN but not diaphragm LECs have intermediate levels of MHC-II We previously showed that LN-LECs express MHC-II molecules [12] . To determine whether this was a specialized property of LN-LECs, we compared the level of MHC-II molecules on LN-LECs with those on tissue lymphatic LECs, other LNSC subsets and haematopoietically derived APC. MHC-II molecules are expressed on LN-LECs, but not on LECs from the diaphragm (D-LECs; Fig. 1a ). LN-LECs express similar levels of MHC-II molecules as LN-BECs and LN-FRCs. Although the geometric mean fluorescence intensity (gMFI) of the entire LEC population is approximately 10% of the gMFI of the entire macrophage population, most LECs express levels of MHC-II similar to that of the lower half of the macrophage profile. This suggests that LECs express levels of MHC-II sufficient for antigen presentation. 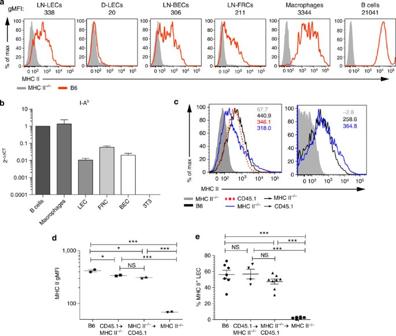Figure 1: LN-LECs endogenously express intermediate levels of MHC-II. (a) Pooled LNs and diaphragms from B6 or MHC-II−/−mice were enzymatically digested. LECs (DAPInegCD45negCD31+gp38+), BECs (DAPInegCD45negCD31+gp38neg), FRCs (DAPInegCD45negCD31neggp38+), macrophages (DAPInegCD11cneg/lowCD11b+F4/80+) and B cells (DAPInegCD19+CD11cnegCD11bneg) were stained extracellularly for MHC-II, and gMFI was calculated. Data representative of at least three experiments with LN pooled from 1 to 2 mice. (b) B cells (DAPInegCD19+), macrophages (DAPInegCD11cneg/lowCD11b+), LECs (DAPInegCD45negCD31+gp38+), FRCs (DAPInegCD45negCD31neggp38+) and BECs (DAPInegCD45negCD31+gp38neg) from B6 mice were sorted by flow cytometry, and cultured 3T3 cells were harvested. Quantitative PCR for I-Abwas performed. Data shown from 2 to 3 independent experiments with LN pooled from 4 to 5 mice. (c–e) Pooled LNs from B6, MHC-II−/−, CD45.1→MHC-II−/−or MHC-II−/−→CD45.1 mice were digested and stained extracellularly for MHC-II expression on LECs. Numbers increpresent gMFI. Representative data (c,d) or cumulative data (e) from 2 to 4 experiments with 1–2 mice each are shown. Groups compared using a one-way analysis of variance with Tukey post-test. *P<0.05; **P<0.01; ***P<0.001, NS=not significant. All data shown as mean±s.e.m. Figure 1: LN-LECs endogenously express intermediate levels of MHC-II. ( a ) Pooled LNs and diaphragms from B6 or MHC-II −/− mice were enzymatically digested. LECs (DAPI neg CD45 neg CD31 + gp38 + ), BECs (DAPI neg CD45 neg CD31 + gp38 neg ), FRCs (DAPI neg CD45 neg CD31 neg gp38 + ), macrophages (DAPI neg CD11c neg/low CD11b + F4/80 + ) and B cells (DAPI neg CD19 + CD11c neg CD11b neg ) were stained extracellularly for MHC-II, and gMFI was calculated. Data representative of at least three experiments with LN pooled from 1 to 2 mice. ( b ) B cells (DAPI neg CD19 + ), macrophages (DAPI neg CD11c neg/low CD11b + ), LECs (DAPI neg CD45 neg CD31 + gp38 + ), FRCs (DAPI neg CD45 neg CD31 neg gp38 + ) and BECs (DAPI neg CD45 neg CD31 + gp38 neg ) from B6 mice were sorted by flow cytometry, and cultured 3T3 cells were harvested. Quantitative PCR for I-A b was performed. Data shown from 2 to 3 independent experiments with LN pooled from 4 to 5 mice. ( c – e ) Pooled LNs from B6, MHC-II −/− , CD45.1→MHC-II −/− or MHC-II −/− →CD45.1 mice were digested and stained extracellularly for MHC-II expression on LECs. Numbers in c represent gMFI. Representative data ( c , d ) or cumulative data ( e ) from 2 to 4 experiments with 1–2 mice each are shown. Groups compared using a one-way analysis of variance with Tukey post-test. * P <0.05; ** P <0.01; *** P <0.001, NS=not significant. All data shown as mean±s.e.m. Full size image We detected mRNA for the I-A b β-chain in C57BL/6 (B6) LECs ( Fig. 1b ), demonstrating that they directly express MHC-II molecules. However, MHC-II molecules can also be acquired from another cell through a process called ‘cross-dressing’ [18] , [19] . We used reciprocal MHC-II −/− bone marrow chimeras to determine the contribution of endogenous synthesis and acquisition from haematopoietically derived cells to the MHC-II molecules displayed by LN-LECs. The LECs in CD45.1→MHC-II −/− bone marrow chimeras continued to display MHC-II molecules, demonstrating they can acquire them from haematopoietically derived cells ( Fig. 1c–e ). However, LECs in the reciprocal MHC-II −/− →CD45.1 chimeras express similar levels of MHC-II molecules. Although there was some heterogeneity between mice ( Fig. 1c , left versus right), the levels of MHC-II and percentages of MHC-II + LECs were similar overall between the two chimera groups ( Fig. 1d,e ). This suggests that the absence of one source of MHC-II molecules is compensated for by another source to maintain a relatively constant level on LECs. These results demonstrate LN-LECs both endogenously synthesize MHC-II molecules and acquire them from haematopoietically derived cells. 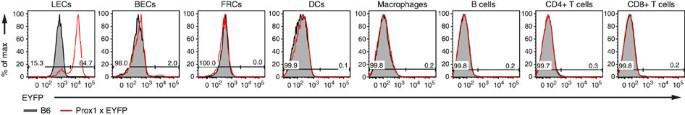Figure 2:Prox1-creERT2is active in LECs but not other LNSCs or haematopoietically derived cells. Prox1-CreERT2x EYFPstop-flox(Prox1xEYFP) mice were maintained on tamoxifen chow for 2 weeks. Pooled inguinal, axillary and brachial LNs from B6 or Prox1xEYFP mice were enzymatically digested and EYFP expression in LECs (DAPInegCD45negCD31+gp38+), BECs (DAPInegCD45negCD31+gp38neg), FRCs (DAPInegCD45negCD31neggp38+), DCs (DAPInegCD11chigh), macrophages (DAPInegCD11cneg/lowCD11b+), B cells (DAPInegCD19+), CD4 T cells (DAPInegCD4+CD19neg) and CD8 T cells (DAPInegCD8+CD19neg) was analysed by flow cytometry. Numbers refer to the percent of EYFP+cells in the Prox1xEYFP mice. Data representative of two independent experiments with 1–2 mice each. Complementary models to evaluate antigen expression in LECs Because there are no CD4 TCR transgenic models directed against endogenous PTAs expressed by LECs, we transgenically expressed β-gal as a model PTA ( Supplementary Table 1 ), as there are β-gal-specific CD4 and CD8 TCR transgenic mice available ( Supplementary Table 2 ). Rosa26 stop-LacZ (ref 20 ) mice express β-gal after cre-mediated excision of a floxed stop cassette. These mice were crossed with mice expressing either Lyve-1-cre [21] or Prox1-creER T2 (ref. 22 ; Supplementary Fig. 1 ). Lyve-1 is used as a specific marker for LECs [23] . Lyve-1-cre is constitutively active in all LECs, and in limited subsets of BECs, lymphoid and myeloid cells [21] . Prox1 is the master transcriptional regulator inducing LEC differentiation [23] . Prox1-creER T2 is induced by tamoxifen, and mediates high-efficiency recombination in LECs but not in BECs, FRCs, DCs, macrophages, B or T cells ( Fig. 2 ). Since Prox1-creER T2 can also lead to recombination in Prox1 + cells in the liver and heart [22] , we used skin-draining LNs in our analysis to eliminate potential effects of antigen draining from these sites. Because these two models, referred to hereafter as Lyve-1xβ-gal and Prox1xβ-gal, differ in their patterns of ectopic expression, they were used as complementary models to investigate LEC-induced tolerance. Figure 2: Prox1-creER T2 is active in LECs but not other LNSCs or haematopoietically derived cells. Prox1-CreER T2 x EYFP stop-flox (Prox1xEYFP) mice were maintained on tamoxifen chow for 2 weeks. Pooled inguinal, axillary and brachial LNs from B6 or Prox1xEYFP mice were enzymatically digested and EYFP expression in LECs (DAPI neg CD45 neg CD31 + gp38 + ), BECs (DAPI neg CD45 neg CD31 + gp38 neg ), FRCs (DAPI neg CD45 neg CD31 neg gp38 + ), DCs (DAPI neg CD11c high ), macrophages (DAPI neg CD11c neg/low CD11b + ), B cells (DAPI neg CD19 + ), CD4 T cells (DAPI neg CD4 + CD19 neg ) and CD8 T cells (DAPI neg CD8 + CD19 neg ) was analysed by flow cytometry. Numbers refer to the percent of EYFP + cells in the Prox1xEYFP mice. Data representative of two independent experiments with 1–2 mice each. Full size image LECs present endogenous β-gal epitopes on MHC-I molecules To determine whether LECs from Lyve-1xβ-gal or Prox1xβ-gal mice express β-gal antigen, we tested whether they activated Bg1 CD8 T cells, which express a transgenic TCR specific for the β-gal 96-103 epitope presented by H-2K b (ref 24 ). A substantial fraction of Bg1 cells proliferated by day 3 after transfer into Prox1xβ-gal mice, and the majority of proliferating cells were gone by day 7 ( Fig. 3a ). As Lyve-1-cre can induce recombination in haematopoietic cells [21] , we used MHC-I −/− →Lyve-1xβ-gal bone marrow chimeras to restrict β-gal expression to radioresistant LNSC. Bg1 cells also proliferated and deleted after adoptive transfer into these mice ( Supplementary Fig. 2a ). In vitro , Bg1 cells proliferated when co-cultured with purified LN-LECs from both models, whereas no significant proliferation was induced by purified FRCs or BECs ( Fig. 3b,c ). Thus, LECs are the only LNSCs in either Lyve-1xβ-gal or Prox1xβ-gal mice that present β-gal 96-103 at immunologically relevant levels. 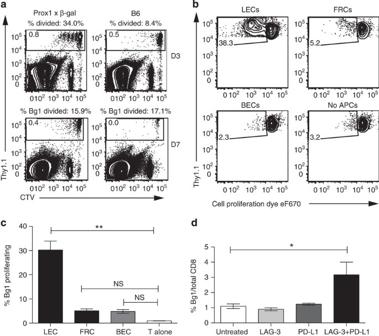Figure 3: LECs induce deletion of β-gal-specific CD8 T cells via the PD-1/PD-L1 and LAG-3/MHC-II pathways. (a) CTV-labelled Thy1.1+Bg1 cells were adoptively transferred along with CTV-labelled Thy1.1negcells as an injection control. Skin-draining LNs were analysed for Bg1 proliferation 3 or 7 days later. Plots are gated on total CD8+T cells. Data representative of 2–3 experiments with 1-3 mice each. LNSCs from Prox1xβ-gal (b) or Lyve-1xβ-gal (c) mice were sorted and co-cultured with Thy1.1+Bg1 T cells for 4 days. Plots are gated on CD8+Thy1.1+Bg1 cells. Data representative of 2–3 experiments with LNs pooled from 4 to 9 mice. Each group was compared with T cells only using a one-way analysis of variance (ANOVA) with Bonferroni post-test. (d) CTV-labelled Thy1.1+Bg1 cells were adoptively transferred along with CTV-labelled Thy1.1negcells as an injection control. Mice were treated with blocking antibodies as described in Methods. Skin-draining LNs were analysed for Bg1 proliferation 7 days later. Data representative of 2 experiments with 1–2 mice each. Treatment groups were compared with untreated group using a one-way ANOVA with Bonferroni post-test. *P<0.05; **P<0.01; NS=not significant. All data shown as mean±s.e.m. Figure 3: LECs induce deletion of β-gal-specific CD8 T cells via the PD-1/PD-L1 and LAG-3/MHC-II pathways. ( a ) CTV-labelled Thy1.1 + Bg1 cells were adoptively transferred along with CTV-labelled Thy1.1 neg cells as an injection control. Skin-draining LNs were analysed for Bg1 proliferation 3 or 7 days later. Plots are gated on total CD8 + T cells. Data representative of 2–3 experiments with 1-3 mice each. LNSCs from Prox1xβ-gal ( b ) or Lyve-1xβ-gal ( c ) mice were sorted and co-cultured with Thy1.1 + Bg1 T cells for 4 days. Plots are gated on CD8 + Thy1.1 + Bg1 cells. Data representative of 2–3 experiments with LNs pooled from 4 to 9 mice. Each group was compared with T cells only using a one-way analysis of variance (ANOVA) with Bonferroni post-test. ( d ) CTV-labelled Thy1.1 + Bg1 cells were adoptively transferred along with CTV-labelled Thy1.1 neg cells as an injection control. Mice were treated with blocking antibodies as described in Methods. Skin-draining LNs were analysed for Bg1 proliferation 7 days later. Data representative of 2 experiments with 1–2 mice each. Treatment groups were compared with untreated group using a one-way ANOVA with Bonferroni post-test. * P <0.05; ** P <0.01; NS=not significant. All data shown as mean±s.e.m. Full size image The loss of proliferating Bg1 cells by day 7 in vivo is consistent with our earlier data demonstrating that LECs induce deletional tolerance. In keeping with this, proliferating Bg1 cells upregulated Annexin V and the inhibitory ligands PD-1 and LAG-3 ( Supplementary Fig. 2b,c ). Although blockade of PD-1/PD-L1 or LAG-3/MHC-II inhibitory pathways individually did not inhibit deletion of Bg1 cells, blockade of both pathways did so ( Fig. 3d and Supplementary Fig. 2d ). This demonstrates that one role for MHC-II molecules on LECs is to promote CD8 T-cell tolerance by engaging LAG-3. LECs do not present endogenous β-gal epitopes on MHC-II To test whether LECs from Prox-1xβ-gal and Lyve-1xβ-gal mice present β-gal epitopes on MHC-II molecules, we used Bg2 CD4 T-cells [25] , which recognize β-gal 721-739 presented by I-A b . Bg2 cells transferred into Lyve-1xβ-gal or Prox-1xβ-gal mice proliferated by day 3 and continued to proliferate and accumulate by day 7 ( Fig. 4a,b ). However, they did not proliferate in MHC-II −/− →Lyve-1xβ-gal or MHC-II −/− →Prox1xβ-gal chimeras, in which radioresistant LECs synthesize MHC-II molecules but bone marrow-derived cells do not. This indicates that Bg2 proliferation in non-chimeric mice is induced by bone marrow-derived cells, but not LECs. We considered that Bg2 T cells might recognize antigen but not proliferate because of the lack of costimulatory molecules on LECs [12] . However, Bg2 cells adoptively transferred into MHC-II −/− →Prox1xβ-gal chimeras treated with αCD28 agonistic antibodies also did not proliferate ( Fig. 4c ). We also considered that LECs might present β-gal, but rapidly induce anergy or suppress T-cell proliferation through nitric oxide [26] , [27] . Therefore, we examined Bg2 cells for upregulation of CD69, CD25 and CD44, and downregulation of CD62L, one day after adoptive transfer. After transfer into non-chimeric Prox1xβ-gal mice, CD69, CD25 and CD44 were all upregulated and CD62L was downregulated ( Fig. 4d ). However, these markers remained unchanged and identical on Bg2 cells transferred into MHC-II −/− →Prox1xβ-gal chimeras and antigen-free B6 mice ( Fig. 4d ), indicating the Bg2 cells were not activated. We conclude that LECs do not present MHC-II-restricted β-gal epitopes to Bg2 cells in vivo , even though they express the source protein and the restriction element. 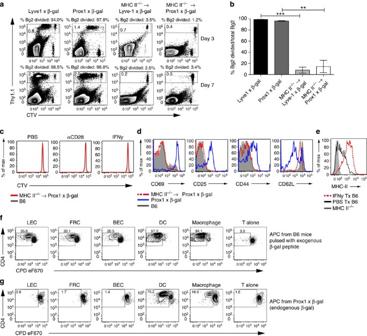Figure 4: LECs do not present endogenous β-gal on MHC-II. (a) Representative and (b) cumulative data of CTV-labelled Thy1.1+Bg2 cells adoptively transferred into the indicated recipients. CTV-labelled Thy1.1negcells were co-transferred as an injection control. Skin-draining LNs were analysed 3 (a) or 7 (a,b) days later, and plots are gated on CD4+T cells. Data representative of 1–3 experiments with 1–4 mice each. Indicated groups were compared using a one-way analysis of variance (ANOVA) with Bonferroni post-test. (c) CTV-labelled Bg2 cells were adoptively transferred into B6 and MHC-II−/−→Prox1xβ-gal mice treated with PBS, αCD28 or IFN-γ, and proliferation was analysed 3 days later. Plots are gated on Thy1.1+CD4+cells. Data representative of 2 experiments with 2 mice each. (d) CTV-labelled Thy1.1+Bg2 cells were transferred into the indicated recipients and activation markers were analysed 16 h later. Plots are gated on Thy1.1+CD4+cells. Data from one experiment. (e) LNs from MHC-II−/−and PBS- or IFN-γ-treated B6 mice were enzymatically digested 24 h after treatment, and MHC-II on LECs was analysed by flow cytometry. Data representative of 3 experiments with 1–2 mice each. (f) LNSCs, DCs and macrophages from B6 mice were sorted by flow cytometry, pulsed with 50 μM Bg2 peptide for 3 h, washed and co-cultured with CPD eF670-labelled Thy1.1+Bg2 T cells for 4 days. (g) LNSCs, DCs and macrophages from Prox1xβ-gal mice were sorted by flow cytometry and co-cultured with CPD eF670-labelled Thy1.1+Bg2 T cells for 4 days. (f,g) Plots are gated on DAPInegCD4+Thy1.1+cells. Data representative of 2 experiments with pooled LNs from 5 to 9 mice. All data shown as mean±s.e.m. Figure 4: LECs do not present endogenous β-gal on MHC-II. ( a ) Representative and ( b ) cumulative data of CTV-labelled Thy1.1 + Bg2 cells adoptively transferred into the indicated recipients. CTV-labelled Thy1.1 neg cells were co-transferred as an injection control. Skin-draining LNs were analysed 3 ( a ) or 7 ( a , b ) days later, and plots are gated on CD4 + T cells. Data representative of 1–3 experiments with 1–4 mice each. Indicated groups were compared using a one-way analysis of variance (ANOVA) with Bonferroni post-test. ( c ) CTV-labelled Bg2 cells were adoptively transferred into B6 and MHC-II −/− →Prox1xβ-gal mice treated with PBS, αCD28 or IFN-γ, and proliferation was analysed 3 days later. Plots are gated on Thy1.1 + CD4 + cells. Data representative of 2 experiments with 2 mice each. ( d ) CTV-labelled Thy1.1 + Bg2 cells were transferred into the indicated recipients and activation markers were analysed 16 h later. Plots are gated on Thy1.1 + CD4 + cells. Data from one experiment. ( e ) LNs from MHC-II −/− and PBS- or IFN-γ-treated B6 mice were enzymatically digested 24 h after treatment, and MHC-II on LECs was analysed by flow cytometry. Data representative of 3 experiments with 1–2 mice each. ( f ) LNSCs, DCs and macrophages from B6 mice were sorted by flow cytometry, pulsed with 50 μM Bg2 peptide for 3 h, washed and co-cultured with CPD eF670-labelled Thy1.1 + Bg2 T cells for 4 days. ( g ) LNSCs, DCs and macrophages from Prox1xβ-gal mice were sorted by flow cytometry and co-cultured with CPD eF670-labelled Thy1.1 + Bg2 T cells for 4 days. ( f , g ) Plots are gated on DAPI neg CD4 + Thy1.1 + cells. Data representative of 2 experiments with pooled LNs from 5 to 9 mice. All data shown as mean±s.e.m. Full size image We next considered that the level of MHC-II on the surface of LECs might be too low to induce CD4 proliferation. In MHC-II −/− →Prox1xβ-gal mice treated with interferon (IFN)-γ, the gMFI of MHC-II on LECs was upregulated more than sixfold ( Fig. 4e ). However, Bg2 cells transferred into these mice also did not proliferate ( Fig. 4c ). Finally, we pulsed FACS-sorted LECs from B6 mice with β-gal 721-739 peptide. Peptide-pulsed LECs induced Bg2 proliferation in vitro ( Fig. 4f ), as did peptide-pulsed FRCs, BECs, DCs and macrophages. The level of proliferation induced by the LNSCs was lower than that induced by DCs, which could reflect lower levels of MHC-II molecules on these cells and/or lack of costimulatory molecules. However, the results demonstrate that the level of MHC-II on LECs is sufficient to present antigen to Bg2 T cells. As LECs were not responsible for the in vivo proliferation of Bg2 cells in non-chimeric Prox1xβ-gal mice ( Fig. 4a ), we used in vitro co-cultures to determine which cells were. LECs, FRCs and BECs sorted by flow cytometry from Prox1xβ-gal mice did not induce Bg2 proliferation ( Fig. 4g ), confirming the in vivo results. However, DCs from these mice induced strong Bg2 proliferation, and macrophages induced a less robust, but still highly significant, response. The basis for antigen presentation by these cells is explored further below. Antigen location does not affect MHC-II presentation in LECs MHC-II presentation of epitopes from cytoplasmic proteins such as β-gal depends on autophagy [28] . Therefore, we investigated whether LECs could present an autophagy-independent I-E d -restricted epitope from the membrane protein influenza HA [29] . We expressed HA in LECs using Prox1-creER T2 x Rosa26 stop-HA (Prox1xHA) (B6 x Balb/c) F1 mice and assessed antigen presentation using HA-specific CD4 or CD8 TCR transgenic cells (TS1 (ref. 30 ) or Clone 4 (ref. 31 ), respectively, also [B6 x Balb/c] F1). LECs from Prox1xHA mice induced proliferation of Clone 4 CD8 T cells in vitro ( Fig. 5a and Supplementary Fig. 3a ), indicating that HA is expressed in LECs and presented on H-2K d MHC-I molecules. However, Prox1xHA LECs did not induce TS1 CD4 T-cell proliferation in vitro ( Fig. 5a and Supplementary Fig. 3a ). A recent report demonstrated that LECs that had acquired peptide:MHC-II complexes from DCs induced CD4 apoptosis in vitro without prior proliferation [19] . However, we saw no difference in death between TS1 cells co-cultured with or without Prox1xHA LECs ( Fig. 5b ). In contrast to LECs, both CD11c + CD11b + and CD11c + CD11b neg DCs presented HA on both MHC-I and MHC-II molecules ( Fig. 5a and Supplementary Fig. 3a ). Corresponding results were seen in vivo , where TS1 cells upregulated CD69 and proliferated in non-chimeric Prox-1xHA mice but not in MHC-II −/− →Prox1xHA chimeras ( Supplementary Fig. 3b,c ). Therefore, like β-gal, HA is presented by LECs on MHC-I molecules, but is not presented on MHC-II molecules. Because Prox1-creER T2 does not induce HA expression in haematopoietic cells, the presentation of HA by two DC subsets indicates that it has been transferred from LECs. 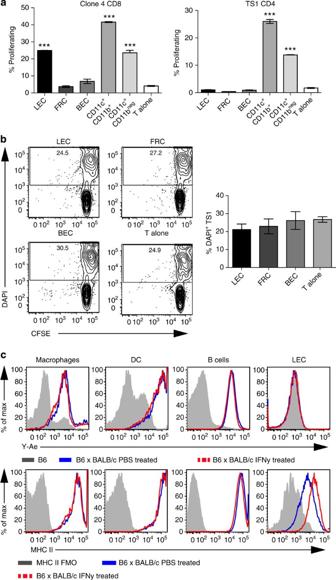Figure 5: LECs do not present MHC-II peptides from the membrane proteins HA and I-Eα. (a,b) LNSCs and DCs from Prox1xHA mice were sorted by flow cytometry and co-cultured with CFSE-labelled Thy1.1+Clone 4 CD8 cells (left) or TS1 CD4 cells (right) for 4 days, and the percent of T cells proliferating was calculated. Each group was compared with T cells alone using a one-way analysis of variance (ANOVA) with Bonferroni post-test. ***P<0.001. Data representative of 2 experiments with LN pooled from 8 mice. (b) The percent of DAPI+TS1 cells from the co-culture inawas calculated. Plots are gated on CD4+Thy1.1+TS1 cells. No significant differences were seen when each group was compared with T cells alone using a one-way ANOVA with Bonferroni post-test. (c) LNs from PBS- or IFN-γ-treated B6 or (B6 x BALB/c) F1 mice were enzymatically digested, and extracellular I-Ab:I-Eα peptide complex expression (top) or MHC-II levels (bottom) were analysed on the indicated populations by flow cytometry. Data representative of 2–3 experiments with 1–3 mice. All data shown as mean±s.e.m. Figure 5: LECs do not present MHC-II peptides from the membrane proteins HA and I-Eα. ( a , b ) LNSCs and DCs from Prox1xHA mice were sorted by flow cytometry and co-cultured with CFSE-labelled Thy1.1 + Clone 4 CD8 cells (left) or TS1 CD4 cells (right) for 4 days, and the percent of T cells proliferating was calculated. Each group was compared with T cells alone using a one-way analysis of variance (ANOVA) with Bonferroni post-test. *** P <0.001. Data representative of 2 experiments with LN pooled from 8 mice. ( b ) The percent of DAPI + TS1 cells from the co-culture in a was calculated. Plots are gated on CD4 + Thy1.1 + TS1 cells. No significant differences were seen when each group was compared with T cells alone using a one-way ANOVA with Bonferroni post-test. ( c ) LNs from PBS- or IFN-γ-treated B6 or (B6 x BALB/c) F1 mice were enzymatically digested, and extracellular I-A b :I-Eα peptide complex expression (top) or MHC-II levels (bottom) were analysed on the indicated populations by flow cytometry. Data representative of 2–3 experiments with 1–3 mice. All data shown as mean±s.e.m. Full size image We also used a T-cell independent assay to directly test whether LECs can form peptide:MHC-II complexes. The Y-Ae antibody recognizes I-A b molecules presenting an epitope derived from the I-Eα chain [32] , which is generated in endosomes [33] . I-Eα, encoded by the H2-Ea-ps gene, was expressed in BALB/c LECs but is a pseudogene and was not expressed in B6 LECs ( Supplementary Fig. 4 ). However, although DCs, macrophages and B cells from (B6 x BALB/c) F1 mice expressed Y-Ae epitopes on the cell surface, LECs did not ( Fig. 5c ). In addition, treating mice with IFN-γ to upregulate I-A b and I-E d did not induce Y-Ae staining on LECs. These results demonstrate that LECs fail to present three separate antigens, which included both cytoplasmic and membrane-bound proteins, and which were restricted by two different MHC-II alleles. Both HA and I-Eα can be presented in the absence of autophagy [29] , [34] , suggesting these results are not due to any impairment of that process in LECs. Instead, the results suggest that there is a fundamental deficiency in the MHC-II processing pathway in LECs. LECs express Ii and Cathepsin L, but not H2-M or H2-O We next investigated whether LECs were deficient in any components of the MHC-II processing pathway. LECs express high levels of Ii ( Fig. 6a ), suggesting that MHC-II molecules are correctly targeted to the MIIC. Ii is degraded by cathepsins S or L, leaving CLIP, which blocks the MHC-II peptide-binding groove. On average, one-third of LAMP1 + endosomes in LECs co-expressed cathepsin L by immunofluorescence microscopy, but there was substantial variation among individual cells and some LN-LECs did not contain detectable Cathepsin L ( Fig. 6b and Supplementary Fig. 5a ). Cathepsin L in LECs was active and cleaved the substrate (CBZ-Phe-Arg) 2 -Rhodamine110 ( Supplementary Fig. 5b ). In contrast, D-LECs did not generate a signal above the background level in cells pretreated with a cathepsin L inhibitor, suggesting that MHC-II neg D-LECs do not express active cathepsin L. The presence of active cathepsin L in some endosomes suggests that LN-LECs can digest Ii into CLIP, although the efficiency of this process may vary among individual cells and endosomes. 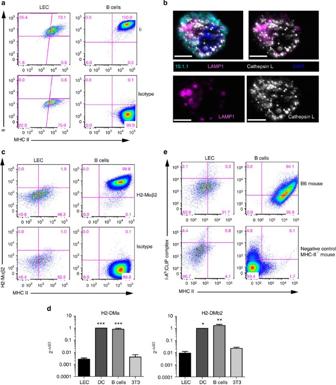Figure 6: LECs express Ii and cathepsin L, but do not express the peptide editor H2-M. (a) B6 LECs (DAPInegCD45negCD31+10.1.1+) and B cells (DAPInegCD19+) were stained intracellularly for Ii and MHC-II or isotype control. The LEC-specific marker 10.1.1 (refs10,12) was used instead of gp38 since 10.1.1 is compatible with intracellular staining protocols. (b) LNs were enzymatically digested, depleted of CD45+cells, stained with 10.1.1 (cyan) extracellularly and cathepsin L (white), LAMP1 (magenta) and DAPI (blue) intracellularly before being cytospun onto slides. Scale bar, 5 μm. (c). LECs and B cells were stained for MHC-II and H2-Mαβ2 intracellularly. (d) LECs, DCs and B cells from B6 mice were sorted by flow cytometry, and 3T3 cells were harvested from culture as inFig. 1. mRNA was purified and quantitative PCR was performed for the indicated genes. LECs were compared with the other groups using a one-way analysis of variance (ANOVA) with Bonferroni post-test. *P<0.05; **P<0.01; ***P<0.001. (e) LECs and B cells from B6 or MHC-II−/−(negative control) mice were stained extracellularly for I-Ab:CLIP complexes and MHC-II. Data ina–c, eare representative of at least 2 experiments with 1–2 mice each, and data indis from 2 experiments with LN pooled from 4 to 5 mice. All data shown as mean±s.e.m. Figure 6: LECs express Ii and cathepsin L, but do not express the peptide editor H2-M. ( a ) B6 LECs (DAPI neg CD45 neg CD31 + 10.1.1 + ) and B cells (DAPI neg CD19 + ) were stained intracellularly for Ii and MHC-II or isotype control. The LEC-specific marker 10.1.1 (refs 10 , 12 ) was used instead of gp38 since 10.1.1 is compatible with intracellular staining protocols. ( b ) LNs were enzymatically digested, depleted of CD45 + cells, stained with 10.1.1 (cyan) extracellularly and cathepsin L (white), LAMP1 (magenta) and DAPI (blue) intracellularly before being cytospun onto slides. Scale bar, 5 μm. ( c ). LECs and B cells were stained for MHC-II and H2-Mαβ2 intracellularly. ( d ) LECs, DCs and B cells from B6 mice were sorted by flow cytometry, and 3T3 cells were harvested from culture as in Fig. 1 . mRNA was purified and quantitative PCR was performed for the indicated genes. LECs were compared with the other groups using a one-way analysis of variance (ANOVA) with Bonferroni post-test. * P <0.05; ** P <0.01; *** P <0.001. ( e ) LECs and B cells from B6 or MHC-II −/− (negative control) mice were stained extracellularly for I-A b :CLIP complexes and MHC-II. Data in a – c, e are representative of at least 2 experiments with 1–2 mice each, and data in d is from 2 experiments with LN pooled from 4 to 5 mice. All data shown as mean±s.e.m. Full size image The peptide editor H2-M exchanges CLIP for antigenic peptides, and also optimizes the repertoire of peptides bound to various MHC-II alleles [35] , [36] , [37] . Its activity is antagonized by H2-O (ref. 17 ). Therefore, low levels of H2-M or high levels of H2-O could explain the inability of LECs to present antigenic peptides. We did not detect either H2-Mαβ2 or H2-O expression in LECs by flow cytometry ( Fig. 6c and Supplementary Fig. 5c ). We also did not detect significant levels of H-2DMα or H-2DMβ2 mRNA ( Fig. 6d ). This suggests that LECs might inefficiently exchange CLIP or suboptimal self-peptides for antigenic peptides. We attempted to measure the level of CLIP bound to I-A b MHC-II molecules using the 15G4 antibody that specifically recognizes I-A b :CLIP complexes. However, background staining in the LEC MHC-II −/− negative control was extremely high, compromising our ability to detect a positive signal in MHC-II +/+ LECs ( Fig. 6e ). With this limitation, our data nonetheless suggest that the most likely explanation(s) for the lack of antigen presentation by LN-LECs are either that Ii associated with MHC-II molecules is not efficiently cleaved into CLIP or that the lack of H2-M prevents the exchange of CLIP or suboptimal self-peptides for optimal antigenic peptides. DCs acquire antigen from LECs to induce anergy Although LECs do not directly present β-gal or HA on MHC-II, these antigens are presented by DCs and macrophages ( Figs 4 and 5 ). As Prox1-creER T2 does not induce genetic recombination in DCs or macrophages ( Fig. 2 ), this indicates that these cells acquired antigen transcribed in LECs. However, antigen presentation did not occur in MHC-II −/− →Prox1xβ-gal ( Fig. 4a–d ) or MHC-II −/− →Prox1xHA ( Supplementary Fig. 3b,c ) chimeras, indicating that antigen is loaded onto MHC-II molecules in haematopoietically derived cells, rather than being transferred as preformed peptide:MHC-II complexes. To formally demonstrate this, we used bone marrow chimeras where genetic expression of β-gal is restricted to either the haematopoietically derived or radioresistant cells. Bg2 cells transferred into Prox-1xβ-gal→CD45.1 chimeras did not proliferate ( Fig. 7a ), demonstrating that β-gal is not genetically expressed in haematopoietically derived cells. In contrast, Bg2 T cells transferred into CD45.1→Prox1xβ-gal chimeras proliferated, confirming that β-gal from LECs is transferred to haematopoietically derived cells. 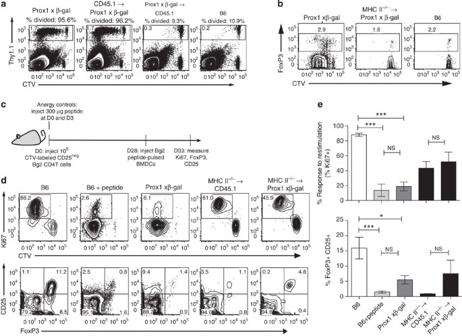Figure 7: Haematopoietically derived cells acquire β-gal from LECs and induce Bg2 anergy. (a) CTV-labelled Thy1.1+Bg2 cells were transferred into the indicated recipients, along with CTV-labelled Thy1.1negcells as an injection control. Proliferation in skin-draining LNs was measured 7 days later. Data representative of 1–2 experiments with 2–5 mice each. (b) CTV-labelled Thy1.1+Bg2 cells were transferred into the indicated recipients, and Tregdevelopment was measured 3 days later. Data representative of 2 experiments with 2–3 mice each. (c) Experimental design to measure tolerance induction. CTV-labelled CD25negThy1.1+Bg2 CD4 T cells were adoptively transferred, and recipient mice were challenged 28 days later with peptide-pulsed BMDCs. Proliferation was measured 5 days later by Ki67 upregulation, and FoxP3 and CD25 were measured to assess Tregformation. (d) Representative and (e) cumulative data gated on CD4+Thy1.1+Bg2 cells from skin-draining LN from 2 experiments with 1–7 mice each. *P<0.05; **P<0.01; ***P<0.001, NS=not significant. Indicated comparisons were made using a one-way analysis of variance with Bonferroni post-test. All data shown as mean±s.e.m. Figure 7: Haematopoietically derived cells acquire β-gal from LECs and induce Bg2 anergy. ( a ) CTV-labelled Thy1.1 + Bg2 cells were transferred into the indicated recipients, along with CTV-labelled Thy1.1 neg cells as an injection control. Proliferation in skin-draining LNs was measured 7 days later. Data representative of 1–2 experiments with 2–5 mice each. ( b ) CTV-labelled Thy1.1 + Bg2 cells were transferred into the indicated recipients, and T reg development was measured 3 days later. Data representative of 2 experiments with 2–3 mice each. ( c ) Experimental design to measure tolerance induction. CTV-labelled CD25 neg Thy1.1 + Bg2 CD4 T cells were adoptively transferred, and recipient mice were challenged 28 days later with peptide-pulsed BMDCs. Proliferation was measured 5 days later by Ki67 upregulation, and FoxP3 and CD25 were measured to assess T reg formation. ( d ) Representative and ( e ) cumulative data gated on CD4 + Thy1.1 + Bg2 cells from skin-draining LN from 2 experiments with 1–7 mice each. * P <0.05; ** P <0.01; *** P <0.001, NS=not significant. Indicated comparisons were made using a one-way analysis of variance with Bonferroni post-test. All data shown as mean±s.e.m. Full size image The presentation of β-gal or HA by haematopoietically derived cells in vivo led to proliferation and accumulation of CD4 T cells over 7 days ( Figs 4a and 7a , and Supplementary Fig. 3c ). To determine the fate of these cells, we tested whether they developed into either T reg or anergic cells. After 3 days, Bg2 cells transferred into Prox1xβ-gal, MHC-II −/− →Prox1xβ-gal and B6 mice all had equivalently low levels of FoxP3 staining ( Fig. 7b ), indicating they were not differentiating into T reg . To test for anergy, we adoptively transferred CD25 neg CTV-labelled Bg2 cells into recipient mice and re-challenged them 28 days later with β-gal 721-739 -pulsed bone marrow-derived DCs (BMDCs). Proliferation was measured 5 days later by Ki67 upregulation ( Fig. 7c ). In this experimental setup, CTV dilute Ki67 pos cells are actively proliferating in response to BMDCs, whereas CTV dilute Ki67 neg cells proliferated initially after adoptive transfer but did not respond subsequently to the β-gal-pulsed BMDCs, and are thus anergic. As expected, Bg2 cells transferred into B6 mice remained naïve and proliferated strongly upon subsequent BMDC stimulation, as evidenced by their dilution of CTV and >85% expression of Ki67 ( Fig. 7d,e ). Consistent with previous work [38] , Bg2 cells transferred into B6 mice treated with 300 μg of β-gal 721 peptide 0 and 3 days after adoptive transfer were CTV dilute and Ki67 neg , and thus anergic. Bg2 cells transferred into Prox-1xβ-gal mice were also CTV dilute Ki67 neg , and therefore were also anergic. Bg2 cells transferred into either MHC-II −/− →Prox-1xβ-gal or control antigen-free MHC-II −/− →CD45.1 bone marrow chimeras were strongly and equivalently CTV dilute Ki67 pos , indicating that anergy does not occur without antigen presentation by haematopoietically derived cells. We also tested whether Bg2 cells differentiate into T reg cells at this later timepoint. We found no increase of FoxP3 + CD25 + Bg2 cells in Prox-1xβ-gal mice compared with B6 mice ( Fig. 7d,e ), further demonstrating that T reg formation is not a form of tolerance induced in this model. These data demonstrate that the antigen transcribed in LECs that is provided to DCs is responsible for anergy induction in CD4 T cells. LECs express a variety of PTAs and directly induce CD8 T-cell tolerance, but their ability to induce CD4 T-cell tolerance to PTAs has not previously been examined. In this study, we demonstrate that MHC-II expression on LECs is sufficient for presentation of exogenously pulsed peptides, but LECs do not present peptides from three endogenous proteins. However, LECs provide antigens to DCs, which then induce anergy. Therefore, LECs serve as a reservoir of PTAs in the LN, which are acquired by DCs for the induction of CD4 T-cell tolerance. In addition, MHC-II plays a role in the deletional tolerance of Bg1 CD8 T-cells, which delete through either the PD-1/PD-L1 or LAG-3/MHC-II pathways after recognizing antigen presented by LECs on MHC-I molecules. LECs do not present epitopes derived from β-gal, HA or I-Eα on their MHC-II molecules. This is independent of antigen source protein localization to the cytoplasm, plasma membrane or endosome, respectively. Because two of these antigens are presented by an autophagy-independent mechanism [29] , [34] , lack of presentation is not due to a defect in autophagy. In addition, the absence of the Y-Ae epitope on LECs suggests that the failure to present is not due to a deficiency in loading source proteins into the MHC-II processing pathway, as I-Eα will be endogenously targeted to the MIIC by Ii as part of the I-E d molecule. LECs express high levels of Ii, suggesting that MHC-II molecules are appropriately chaperoned into the MIIC. In addition, cathepsin L is active and expressed in a subset of LEC LAMP-1 + endosomes. This suggests that Ii can be cleaved into CLIP in many cells, but it is also possible that MHC-II molecules maturing in cathepsin L neg endosomes contain Ii instead of CLIP. However, LECs also do not express H2-M, suggesting that even if CLIP is generated it may be inefficiently exchanged for antigenic peptides. Unfortunately, a high level of nonspecific background CLIP staining in LECs prevented direct evaluation of this latter hypothesis. It has been shown that for MHC-II alleles with a relatively low affinity for CLIP, competition from non-optimal endogenous peptides in the absence of H2-M can limit effective presentation of exogenous epitopes [35] , [36] , [37] . Consistent with this, Y-Ae expression and presentation of HA 109-119 on I-E d are both dependent on H2-M [39] , [40] . Thus, lack of MHC-II-restricted epitope presentation by LECs is likely due to deficiencies in expression of H2-M, and potentially that of cathepsin L as well. Although class II transactivator (CIITA) usually drives co-expression of MHC-II, Ii and H2-M, several papers have shown that MHC-II [41] , [42] , [43] , [44] , [45] , [46] , [47] and invariant chain [48] can be expressed independently of CIITA, and invariant chain can be expressed independently of MHC-II [49] . CIITA-independent transcription of MHC-II molecules in endothelial cells has also been described [44] . Most importantly, kidney glomerular endothelial cells have been shown to express HLA-DR MHC-II molecules in the absence of the human homologue of H2-M, HLA-DM [50] . However, the mechanism(s) of this differential regulation have not been defined. Alternatively, H2-M mRNA could be degraded in LECs by microRNA, preventing translation. It is interesting to speculate that MHC-II molecules may be expressed independently of H2-M as a means to separate the generation of a LAG-3 ligand from generation of antigens. Although the transcriptional mechanisms used in LECs to induce MHC-II molecules and Ii in the absence of H2-M remain to be determined, our data suggest that the most likely model is that MHC-II:Ii complexes are correctly targeted into the MIIC, but antigenic peptides are inefficiently loaded for presentation due to a lack of H2-M and possibly inefficient Ii cleavage by cathepsin L. Our work demonstrating a lack of endogenous antigen presentation by LECs is relevant to three other recently published studies. Onder et al. [51] used podoplanin-cre transgenic mice to induce β-gal expression in FRCs and LECs, analogous to our models, and saw in vivo proliferation of Bg2 cells transferred into these mice. However, they did not evaluate the cell populations that presented antigen. Our results suggest that their observations were due to antigen transfer from LECs to DCs and macrophages, rather than direct presentation by either FRCs or LECs. In a second study, Dubrot et al. [19] showed that LECs acquired preloaded peptide:MHC-II complexes from DCs and directly induced apoptosis of antigen-specific T cells in vitro in the absence of proliferation [19] . Our data support their conclusion that LECs can acquire MHC-II molecules from haematopoietic cells through cross-dressing. However, we also found that LECs synthesize a large fraction of the MHC-II molecules that they express. Importantly, our results establish that LECs provide source proteins to DCs for efficient presentation by both MHC-I and MHC-II molecules. However, in contrast to Dubrot et al. , we saw no evidence that these particular MHC-II:peptide complexes were transferred back to the LECs in vivo in sufficient quantities to induce CD4 T-cell recognition, either in vitro or in vivo . Thus, our results argue against a general role for LECs in tolerance induction through presentation of cross-dressed MHC-II molecules acquired from DCs. One possible explanation for the difference between our study and theirs is that Dubrot et al. used an antigen genetically expressed in DCs, potentially expanding the amount of antigen available as well as the number of DCs expressing it, which may have increased the level of cross-dressed antigen:MHC-II complexes to unusually high levels. However, they did not specifically demonstrate CD4 T-cell recognition of antigens displayed on MHC-II by LECs in vivo , and the form of apoptotic death demonstrated in vitro was unusual. It is clear that much remains to be done to establish the relevance of LEC cross-dressing for in vivo tolerance induction. A third study recently published by Baptista et al. [52] showed that the transplantation of MHC-II neg LN (and thus MHC-II neg LNSCs) into wild-type mice reduces the frequency of T reg cells and increases CD4 and CD8 T-cell activation, suggesting that one or more LNSC populations present antigens on MHC-II. Although LECs were not specifically evaluated, an alternative explanation not explored in this paper is that the effect could be due to loss of the LAG-3/MHC-II pathway. This pathway has been shown to enhance T reg function and inhibit T-cell effector activity [15] , [53] , and our work demonstrates that LECs use it for the induction of CD8 T-cell tolerance. In addition, Baptista et al. [52] elegantly demonstrate that transplantation of OVA + LNs induces tolerance to delayed type hypersensitivity and skin transplantation. However, they do not investigate whether this was due to direct antigen presentation by LNSCs, or to antigen acquisition and presentation by CD45 + haematopoietic cells. As our work shows that CD45 + cells can induce tolerance using antigen acquired from LECs, this mechanism also needs to be considered. Our results provide compelling evidence that LECs indirectly function in peripheral CD4 tolerance by serving as a reservoir of PTAs in the LN, which are acquired and presented by DCs to induce anergy. Similarly, mTECs and DCs share responsibility for CD4 tolerance induction in the thymus. mTECs express high levels of MHC-II, and directly present some antigens to CD4 T cells, whereas others are transferred to DCs [1] , [54] , [55] , [56] , [57] , [58] , [59] . It is unclear what determines whether an antigen is presented by mTECs, DCs or both. mTECs are not highly phagocytic [60] , but do constitutively undergo autophagy [34] , and disrupting autophagy shifts presentation of a model antigen from mTECs to DCs [61] . Thus, one model is that PTAs not efficiently incorporated into autosomes are presented by DCs instead of mTECs. Although it is unknown whether LECs constitutively undergo autophagy, presentation of HA and I-Eα on MHC-II molecules does not require autophagy [29] , [34] , suggesting this alone would not preclude presentation. Our work demonstrates LECs transfer PTAs to DCs for the induction of tolerance, a process analogous to that occurring in the thymus. Interestingly, a recent report demonstrated that viral antigens are archived in LECs and subsequently transferred to DCs for the maintenance of memory T-cells and enhanced protective immunity [62] . This indicates extensive cross-talk between LECs and DCs in the LN, and future studies may determine how tolerogenic versus immunogenic antigens are separated in LECs and transferred to DCs. A variety of different mechanisms are used to transfer antigens among different cell types. Gut macrophages transfer antigens to CD103 + DCs through gap junctions during oral tolerance [63] . Antigen transfer can also occur through exosomes [64] or phagocytosis of apoptotic cells [65] , [66] . Transfer of peptide:MHC-II complexes from DCs to LECs occurs through cell contact and/or exosomes [19] . LECs could potentially transfer antigens to DCs through exosomes, gap junctions or DC phagocytosis of apoptotic LECs. We found that transfer of β-gal from LECs to DCs does not solely rely on phagocytosis, as blocking phosphatidylserine recognition or inhibiting DC phagocytosis does not block antigen transfer in vivo (unpublished data). Although the CD11b + CD11c + DC subset is generally considered to be specialized for antigen presentation to CD4 T cells and CD11b neg CD11c + DCs are specialized for antigen presentation to CD8 T cells [7] , we found that HA is presented to CD4 and CD8 T cells by both CD11b neg CD11c + and CD11b + CD11c + DC subsets. This suggests that HA is non-specifically acquired and presented by multiple subsets of DCs. Further work is needed to elucidate the exact mechanism by which PTAs are transferred from LECs to DCs. Although MHC-II molecules on LECs do not directly present peptides for CD4 T-cell tolerance, they play an important role in CD8 T-cell tolerance. We previously demonstrated LECs induce deletion of tyrosinase-specific CD8 T cells through PD-1/PD-L1 (ref. 12 ). Here, we show that both the PD-1/PD-L1 and LAG-3/MHC-II pathways are used in combination to tolerize β-gal-specific CD8 T cells. LAG-3 and PD-1 act synergistically in other tolerance models [15] . Although we have not specifically shown that MHC-II on LECs is used as the ligand for LAG-3, this is likely as LECs are the only cells presenting β-gal 96-103 in MHC-I −/− →Lyve-1xβ-gal bone marrow chimeras. Our results demonstrate that LECs use multiple inhibitory pathways to enforce CD8 T-cell tolerance. In summary, we have demonstrated that although LN-LECs express intermediate levels of MHC-II molecules, they do not present MHC-II β-gal, HA or I-Eα peptides. Instead, MHC-II is important to enforce CD8 T-cell tolerance through the LAG-3 pathway. LECs indirectly induce CD4 anergy by transcribing PTAs and transferring them to DCs for MHC-II presentation, a process analogous to what occurs in the thymus. As thymic tolerance is incomplete, peripheral transcription of PTAs by LECs ensures that self-reactive T cells have multiple opportunities to be tolerized. By directly inducing CD8 T-cell deletion as well as transferring antigens to DCs for CD4 anergy, LECs play multiple tolerogenic roles. Mice C57Bl/6 (B6) and CD45.1 (B6-LY5.2/Cr) were from NCI. MHC-II −/− (B6.129- H2-Ab1 tm1Gru N12) and MHC-I −/− (B6.129P2- H2-Kb tm1 H2-Db tm1 N12) [67] mice were from Taconic (NIAID Exchange Program). Lyve-1-cre ( B6;129P2-Lyve1 tm1.1(EGFP/cre)Cys /J ) [21] , β-gal (B6.129S4- Gt(ROSA)26Sor tm1Sor /J) [20] , EYFP (B6.129X1- Gt(ROSA)26Sor tm1(EYFP)Cos /J) and Clone 4 (CBy.Cg-Thy1a Tg(TcraCl4,TcrbCl4)1Shrm/ShrmJ, Jax) [31] mice were from Jax. Bg1 (ref. 24 ) and Bg2 (ref. 25 ) mice from Christopher Norbury (Pennsylvania State University) were crossed to Thy1.1 mice (Jax). Prox1-creERT2 (ref. 22 ) and Rosa26 tm(HA)1Libl mice [68] have been described. TS1 (ref. 30 ) mice were from Andrew Caton (University of Pennsylvania). All mice other than Clone 4, Clone 6.5 and Rosa26 tm(HA)1Libl are on a B6 background. The BALB/c Clone 4 and Clone 6.5 mice were crossed to B6 Thy1.1 mice, and the resulting (BALB/c x B6) background mice were used for adoptive transfers into Prox1-creER T2 x Rosa26 tm(HA)1Libl (BALB/c x B6) recipients. Prox1-creER T2 was induced with tamoxifen chow (TAM400, Harlan) for 2 weeks before experiments, and mice were maintained on TAM400 throughout the course of the experiment. Male and female mice were used between the ages of 6 and 32 weeks. Animals were maintained in pathogen-free facilities. This study was carried out in strict accordance with the recommendations in the Guide for the Care and Use of Laboratory Animals of the National Institutes of Health. Procedures were approved by the University of Virginia Animal Care and Use Committee. LNSC and DC isolation LNs (pooled inguinal, axillary, brachial, cervical and mesenteric) were digested for 45–60 min at 37 °C using 0.42 U ml −1 Liberase TM (Roche) and 60 U ml −1 DNase I (Sigma) in DMEM (Cellgro) with 2% FCS, essential and non-essential amino acids, sodium pyruvate and HEPES. Red blood cells were lysed (Sigma). CD45 + cells were labelled with CD45 magnetic beads in AwesomeMACS (PBS with 0.5% BSA, 2 mM EDTA, 2 mM L-glutamate, 10 mM sodium pyruvate, 1 × essential and non-essential amino acids, and 4.5 g l −1 dextrose) and separated using the Deplete AutoMACS protocol (Miltenyi Biotec). For in vitro co-cultures, DCs and macrophages were enriched using CD11c + and CD11b + beads (Miltenyi Biotec) before CD45 depletion. Cells were stained andanalysed by flow cytometry (see below), or sorted by flow cytometry using Influx (BD), FACSVantage (BD) or iCyt Reflection (Sony) cell sorters for in vitro co-cultures and quantitative PCR. In vitro co-culture Antigen-specific T cells were enriched using CD4 or CD8 magnetic beads (Miltenyi Biotec) and labelled with 1 μM carboxyfluorescein succinimidyl ester (CFSE) or cell proliferation dye eF670 (CPD eF670, eBioscience). T cells were co-cultured with FACS-sorted LNSCs, DCs or macrophages at a 1:2 (T-cell/APC) ratio for 4 days in RPMI-1640 with 10% FCS, 2 mM L-glutamine, 30 mM HEPES, 10 mM sodium pyruvate, 0.05 mM β-mercaptoethanol, 1 × essential and non-essential amino acids, and 0.05 mg ml −1 gentamycin containing IL-2 (10 U ml −1 ) and IL-7 (1 pg ml −1 for CD8 T cells and 1 ng ml −1 for CD4 T cells). CD4 co-cultures also received 0.25 μg ml −1 αCD28 (clone 37.51). Adoptive transfer Thy1.1 + antigen-specific T cells were positively selected with CD4 or CD8 beads or CD25 neg CD4 + cells were negatively selected using a regulatory T-cell isolation kit (Miltenyi Biotec). Cells were labelled with Cell Trace Violet (CTV, Invitrogen), and 1 × 10 6 antigen-specific T cells were injected intravenously. Thy1.2 + CTV-labelled congenic cells were used as an injection control. Skin-draining LN (inguinal, axillary, brachial) were harvested from recipient mice 1, 3, 7 or 33 days after adoptive transfer. In vivo antibody and IFN-γ treatment Mice were injected with 100 μg anti-CD28 (clone 37.51, BioXCell) IP at days 0 and 2. 100 μg anti-LAG-3 (C9B7W, BioXCell) and/or anti-PD-L1 (10B5, University of Virginia Lymphocyte Culture Center or BioXCell) were injected intraperitoneally (IP) at days −1, 1, 3 and 5. IFN-γ (5 × 10 4 U, Peprotech) was injected intravenously (IV) at days −1 and 1 for adoptive transfer experiments, and 24 h before harvest for Y-Ae staining experiments. Mice were randomly assigned to treatment groups. Bone marrow chimeras Mice were irradiated (6.5 Gy × 2) and reconstituted with a minimum of 2 × 10 6 bone marrow cells depleted of CD4 + and CD8 + T cells (Miltenyi Biotec) to prevent graft-versus-host disease. Chimeras were maintained on sulfa water for 3 weeks, and allowed to reconstitute for at least 8 weeks before use. Flow cytometry Antibodies used include: Ii (In-1, 1:100), H2-M (2E5A, 1:50), Rat IgG1 (R3-34, 1:50; all from BD Biosciences); podoplanin (8.1.1, BioLegend, 1:500); CLIP (15G4, Santa Cruz, 1:5); H2-O (ref. 69 ; Mags.Ob3, Lisa Denzin, 1:400); 10.1.1 (UVA lymphocyte culture centre, 1:1,000); CD45 (30-F11, 1:1,000), CD31 (390, 1:1,000), MHC-II (M5/114.15.2, 1:50 ( Fig. 1 ) to 1:500 ( Fig. 6 )), CD8 (53-6.7, 1:1,000), CD4 (GK1.5, 1:1,000), Thy1.1 (HIS51, 1:1,000), Thy1.2 (53-2.1, 1:1,000), CD45.1 (A20, 1:500), CD11c (N418, 1:500), CD11b (M1/70, 1:500), CD69 (H1.2F3, 1:500), CD62L (MEL-14, 1:1,000), CD44 (IM7, 1:1,000), CD25 (PC61.5, 1:500), Y-AE (eBioY-Ae, 1:200), PD-1 (RMP1-30, 1:100), LAG-3 (eBioC9B7W, 1:100), Rat IgG2b (eB149/10H5; all from eBioscience). Intracellular staining for PD-1, LAG-3, Ii, H2-M and H2-O was done using the Cytofix/Cytoperm kit (BD Bioscience), and Ki67 (SolA15, 1:500) and FoxP3 (FJK-16s, 1:100) were stained using Treg permeabilization buffers (eBioscience). Annexin V (1:20) was stained using the eBioscience kit. 4,6-Diamidino-2-phenylindole (DAPI; Sigma) or live/dead aqua (Invitrogen, 1:200) were used to distinguish live cells. Cells were acquired on a FACSCanto II (BD Biosciences) and data analysed using FlowJo (Tree Star). Cathepsin L assay LN-LECs or D-LECs were preincubated with 1 mM of the cathepsin L inhibitor 1-naphthalenesulfonyl-IW-CHO (Calbiochem) or dimethylsulphoxide vehicle control for 20 min at 37 °C, followed by a 20-min incubation with 50 μM of the cathepsin L substrate (CBZ-Phe-Arg) 2 -rhodamine 110 (Invitrogen) at 37 °C before being acquired on a FACSCanto II. Immunofluorescence microscopy LNs were enzymatically digested, depleted of CD45 + cells, stained with 10.1.1 extracellularly and CD107a (1D48, BioLegend), cathepsin L (EPR8011, Abcam), biotin-anti-rabbit (Vector labs) and streptavidin Dylite 550 (Thermo Scientific) intracellularly before being cytospun onto slides and mounted with Slow Fade Gold with DAPI. Images were taken using an Axio Imager 2 with Apotome (Carl Zeiss), and brightness and contrast were adjusted using Zen software (Carl Zeiss). LAMP1 and cathepsin L co-localization Single colour images of LAMP1 and cathepsin L staining were imported into ImageJ and thresholded to identify positive vesicles as greater than 10 pixels in area. The percent of these vesicles co-expressing cathepsin L per cell was measured. Histograms were computed using GraphPad Prism. Quantitative PCR Cells were sorted by flow cytometry into RNA Protect (Qiagen). mRNA was purified using either the RNeasy Mini or Plus Micro kits (Qiagen), and cDNA was synthesized using the iScript cDNA synthesis kit (Bio-Rad). Amplification of I-Ab ( H2-Ab1 ), H2-Mα, H2-DMβ2 and HPRT was performed using iQ SYBR Green Supermix (Bio-Rad) and amplification of I-Eα and HPRT was performed using TaqMan Master Mix (Life Technologies) on a MyiQ qPCR Detection System (Bio-Rad). SYBR Green reactions were run at 95 °C for 10 min followed by 40 cycles of 95 °C for 30 s and 60 °C for 1 min. TaqMan reactions were run at 50 °C for 2 min, 95 °C for 10 min and 40 cycles of 95 °C for 15 s and 60 °C for 1 min. Primers used were the following: Hprt forward, 5′-AGGTTGCAAGCTTGCTGGT-3′, and reverse, 5′-TGAAGTACTCATTATAGTCAAGGGCA-3′; H2-Ma forward, 5′-CTCGAAGCATCTACACCAGTG-3′, and reverse, 5′-TCCGAGAGCCCTATGTTGGG-3′; H2-DMb2 forward, 5′-GTTGGCTTCTTCAGATGGCG-3′, and reverse, 5′-TGCCGTCCTTCTGGGTAGG-3′; H2-Ab1 forward, 5′-GGTGTGCAGACACAACTACG-3′, and reverse, 5′-CGACATTGGGCTGTTCAAGC. Taqman probes (Life Technologies) used were Mm00446968_m1 for HPRT and Mm00772352_m1 for H2-Ea-ps (I-Eα). Ct values were normalized to HPRT and relative expression compared with B cells or dendritic cells was reported as 2 −ΔΔCt . BMDCs Bone marrow cells were isolated from the tibias and femurs of B6 mice, cultured in vitro in RPMI-1640 with 10% FCS, 2 mM L -glutamine, 30 mM HEPES, 0.05 mM β-mercaptoethanol and 0.05 mg ml −1 gentamycin, supplemented with 1,000 U ml −1 GM-CSF (BD Biosciences) and 100 U ml −1 IL-4 (eBioscience). Medium was changed on day 2 and the top half of the medium was changed on day 5 of culture. On day 7, BMDCs were harvested, enriched for CD11c + cells (Miltenyi Biotec) and activated overnight with NIH 3T3 cells expressing CD40L [70] (provided by R. Lapoint, University of Montreal). Activated BMDCs were pulsed with 50 μg ml −1 of β-gal 721-739 (AENLSVTLPAASHAIPHLT, GenScript) for 3 h, washed and 1 × 10 5 BMDCs were injected IV. Statistical analysis Statistical analysis of data was performed using GraphPad Prism 5. P values <0.05 were considered statistically significant; * P <0.05; ** P <0.01; *** P <0.001, NS=not significant. Two-tailed unpaired t -tests were used for comparisons between two groups, and a one-way analysis of variance with Tukey or Bonferroni post-test was used for three or more groups. All data shown as mean±s.e.m. How to cite this article: Rouhani, S. J. et al. Roles of lymphatic endothelial cells expressing peripheral tissue antigens in CD4 T-cell tolerance induction. Nat. Commun. 6:6771 doi: 10.1038/ncomms7771 (2015).